Crystal structure of human tyrosylprotein sulfotransferase-2 reveals the mechanism of protein tyrosine sulfation reaction Post-translational protein modification by tyrosine sulfation has an important role in extracellular protein–protein interactions. The protein tyrosine sulfation reaction is catalysed by the Golgi enzyme called the tyrosylprotein sulfotransferase. To date, no crystal structure is available for tyrosylprotein sulfotransferase. Detailed mechanism of protein tyrosine sulfation reaction has thus remained unclear. Here we present the first crystal structure of the human tyrosylprotein sulfotransferase isoform 2 complexed with a substrate peptide (C4P5Y3) derived from complement C4 and 3′-phosphoadenosine-5′-phosphate at 1.9 Å resolution. Structural and complementary mutational analyses revealed the molecular basis for catalysis being an S N 2-like in-line displacement mechanism. Tyrosylprotein sulfotransferase isoform 2 appeared to recognize the C4 peptide in a deep cleft by using a short parallel β-sheet type interaction, and the bound C4P5Y3 forms an L-shaped structure. Surprisingly, the mode of substrate peptide recognition observed in the tyrosylprotein sulfotransferase isoform 2 structure resembles that observed for the receptor type tyrosine kinases. Post-translational protein modification by tyrosine sulfation, first discovered in bovine fibrinogen [1] , is now known to have a widespread occurrence among proteins in multicellular eukaryotic organisms [2] , [3] . While the functional involvement of protein tyrosine sulfation remains to be fully elucidated, it has been implicated in the alteration of biological activity of proteins, proteolytic processing of bioactive peptides [4] , change in half-life of proteins in circulation [5] , and modulation of extracellular protein–protein interactions including inflammatory leucocyte adhesion [6] , [7] . The recent discovery of the tyrosine sulfation of chemokine receptors suggests an even broader role in inflammatory response [8] , [9] . In the case of the chemokine receptor CCR5, the sulfated tyrosine residues located in its N-terminal extracellular region have been shown to be crucial in mediating HIV binding/infection [10] , [11] , [12] . Tyrosylprotein sulfotransferases (TPSTs) catalyse the transfer of a sulphonate moiety from 3′-phosphoadenosine-5′-phosphosulfate (PAPS) to the hydroxyl group of protein-bound tyrosine residue to form a tyrosine O -sulphate ester and 3′-phosphoadenosine-5′-phosphate (PAP) ( Fig. 1a ). TPSTs are integral membrane glycoproteins located in the trans -Golgi network [2] . In humans, two TPST isoforms, designated TPST1 and TPST2, have been identified [13] , [14] , [15] . The two enzymes consist of 370 and 377 amino-acid residues, respectively, sharing 64% amino-acid sequence identity ( Supplementary Fig. S1 ). They have been shown to display slightly different substrate specificities [16] . Both TPST1 and TPST2 have the type II transmembrane topology with a short N-terminal cytoplasmic domain, a single 17-residue transmembrane domain, and a putative stem region of about 40 residues, followed by a luminally oriented catalytic domain [14] , [15] . 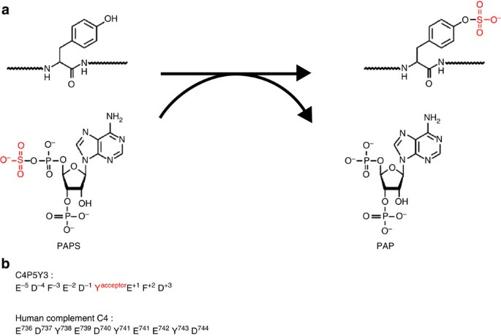Figure 1: Post-translational tyrosine sulfation reaction as catalysed by TPST. (a) The tyrosine residue of a substrate protein is sulfated by TPST using the sulphate donor, PAPS. (b) The amino-acid sequences of substrate peptides used in this study. The C4P5Y3 peptide is derived from a region encompassing a sulfation site (Y741) in human complement C4. F−3and F+2residues of C4P5Y3 correspond to tyrosine residues (Y738 and Y743, respectively) in complement C4 protein. Figure 1: Post-translational tyrosine sulfation reaction as catalysed by TPST. ( a ) The tyrosine residue of a substrate protein is sulfated by TPST using the sulphate donor, PAPS. ( b ) The amino-acid sequences of substrate peptides used in this study. The C4P5Y3 peptide is derived from a region encompassing a sulfation site (Y741) in human complement C4. F −3 and F +2 residues of C4P5Y3 correspond to tyrosine residues (Y738 and Y743, respectively) in complement C4 protein. Full size image Previous studies indicated that TPSTs recognize accessible tyrosine residues that are usually surrounded by several acidic residues within −5 to +5 positions [17] , [18] . However, no general consensus sequence for tyrosine sulfation sites has been defined. Furthermore, because no structure of TPST was available, the mechanisms by which the TPSTs recognize their protein substrates and catalyse the sulfation reaction had remained unclear. Here we present the first crystal structure of the human TPST isoform 2 (TPST2) complexed with C4P5Y3, a substrate peptide derived from complement C4, and PAP at 1.9 Å resolution. Structural and complementary mutational analyses revealed the molecular basis for both catalysis and substrate peptide recognition. Crystal structure of human TPST2 A crystal structure of a proteolytically defined 38-kDa core domain of human TPST2 (designated TPST2ΔC18; encompassing Gly43-Leu359 of TPST2), complexed with PAP and C4P5Y3, was solved at a resolution of 1.9 Å. The C4P5Y3 peptide corresponds to a nine-amino-acid region encompassing the tyrosine sulfation site (Y741) of human complement C4 ( Fig. 1b ). This peptide, E −5 -D −4 -F −3 -E −2 -D −1 -Y acceptor -E +1 -F +2 -D +3 (Y acceptor represents the acceptor site for sulfation), had been reported to be sulfated by the rat TPST with a K m of 5.4 μM (ref. 19 ). (Two Tyr residues (Y738 and Y743) in the original sequences have been mutated to Phe (F) and only one Tyr (Y741) residue exists in the peptide.) The TPST2ΔC18 catalytic domain comprises a single α/β motif with a five-stranded parallel β-sheet, flanked on both sides by α helices ( Fig. 2a ). Central to this structural motif is the 5′-phosphosulfate-binding (5′-PSB) motif (75-GVPRSGTTL-83), contained within a strand-loop-helix consisted of β3 and α1 ( Supplementary Figs S2 and S3a ). This loop can form extensive interactions with the 5′-phosphosulfate of PAPS. Moreover, β6 and α7 are also key elements that include the 3′-phosphate-binding (3′-PB) motif of PAPS ( Supplementary Figs S2 and S3a ). The 5′-PSB and 3′-PB motifs are known to be conserved among all members of the sulfotransferase family [20] , [21] . The arrangement of these secondary structures is very similar in structure to the P-loop found in some kinases such as UK as described in a previous report on SULT1E1 [20] . 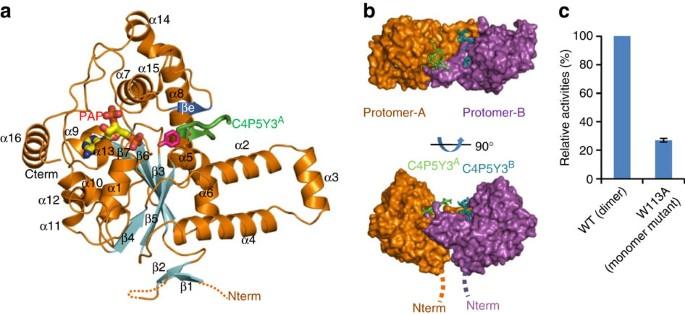Figure 2: The crystal structure of TPST2ΔC18 in complex with PAP and C4P5Y3 peptide. (a) One protomer ribbon diagram of the TPST2ΔC18-PAP (yellow)-C4P5Y3 peptide (green) ternary complex. α-helices and β-strands are coloured orange and cyan, respectively. The TPST2ΔC18 catalytic domain comprises a single α/β motif with a five-stranded parallel β-sheet (β7-β6-β3-β5-β4) flanked on both sides by α-helices. Three consecutive α-helices (α2, α3 and α4) protrude from the roughly spherical configuration of the TPST2ΔC18. (b) Dimeric complex of the core domain of TPST2ΔC18. The lower diagram shows the side view of the dimer (protomer A and B are coloured orange and purple, respectively). The hypothetical positions of the N termini of both protomers have been sketched into the figure. The Golgi membrane is located ipsilateral to the N-termini. The upper diagram shows the view of the TPST2ΔC18 dimer looking down the homodimer two-fold axis. The dimeric complex has two active sites and binds two C4P5Y3 peptides. To distinguish between the two bound C4P5Y3 peptides, the peptides sulfated by A-protomer and B-protomer are referred to as C4P5Y3Aand C4P5Y3B, respectively. The diagrams shown in the figure were prepared using PyMol (http://pymol.sourceforge.net). (c) Site-directed mutagenesis study was performed to probe the role of W113 in dimer interface of TPST2. Sulfotransferase activity assay was performed using C4P5Y3 as the substrate peptide. The blue bar graph illustrates the relative activities of different mutant TPST2s, compared with that of the wild-type TPST2 as 100%.n=3, mean±s.e.m. Figure 2: The crystal structure of TPST2ΔC18 in complex with PAP and C4P5Y3 peptide. ( a ) One protomer ribbon diagram of the TPST2ΔC18-PAP (yellow)-C4P5Y3 peptide (green) ternary complex. α-helices and β-strands are coloured orange and cyan, respectively. The TPST2ΔC18 catalytic domain comprises a single α/β motif with a five-stranded parallel β-sheet (β7-β6-β3-β5-β4) flanked on both sides by α-helices. Three consecutive α-helices (α2, α3 and α4) protrude from the roughly spherical configuration of the TPST2ΔC18. ( b ) Dimeric complex of the core domain of TPST2ΔC18. The lower diagram shows the side view of the dimer (protomer A and B are coloured orange and purple, respectively). The hypothetical positions of the N termini of both protomers have been sketched into the figure. The Golgi membrane is located ipsilateral to the N-termini. The upper diagram shows the view of the TPST2ΔC18 dimer looking down the homodimer two-fold axis. The dimeric complex has two active sites and binds two C4P5Y3 peptides. To distinguish between the two bound C4P5Y3 peptides, the peptides sulfated by A-protomer and B-protomer are referred to as C4P5Y3 A and C4P5Y3 B , respectively. The diagrams shown in the figure were prepared using PyMol ( http://pymol.sourceforge.net ). ( c ) Site-directed mutagenesis study was performed to probe the role of W113 in dimer interface of TPST2. Sulfotransferase activity assay was performed using C4P5Y3 as the substrate peptide. The blue bar graph illustrates the relative activities of different mutant TPST2s, compared with that of the wild-type TPST2 as 100%. n =3, mean±s.e.m. Full size image Dimer interface Previous studies suggested that TPST enzymes exist as dimeric proteins that are formed primarily through the interaction of the transmembrane segments of the two constituent subunits [15] , [22] . Interestingly, although the transmembrane segment is not present, the 38-kDa core domain of TPST2ΔC18 still forms a homodimer (with the two subunits designated, respectively, as protomers A and B) as mediated by three consecutive α-helices (α2, α3 and α4) ( Fig. 2b and Supplementary Fig. S3a ). The dimer interface buries ~25% of the surface area of each protomer. The orientation of the protomers positions the N termini of both subunits on one side of the dimer and in close proximity to each other ( Fig. 2b ). This orientation is consistent with a type II membrane-bound protein where both subunits would be anchored to the membrane via their N-terminal transmembrane domains. That the TPST2ΔC18 core domain exists as a dimer was further supported by results from gel filtration chromatography ( Supplementary Fig. S4a ). TPST2ΔC18 was eluted with a calculated molecular mass of ~77 kDa, consistent with that of a dimeric molecule. Additionally, a low-resolution TPST2 (Gly43-Ser377)-PAP binary complex structure without C4 peptides, belonging to a different space group ( P 22 1 2 1 ), also showed a similar dimeric structure ( Supplementary Fig. S4b ). The dimerization results in the formation of the acceptor–substrate binding sites in both protomers. Although no disulphide bond is present between the protomers in either of the two crystal structures, C31, which is not included in crystallized regions, is present immediately after transmenbrene domain. Therefore, it is possible that C31 could be involved in homodimer formation in the full-length enzyme. The dimer formation mediated by the three consecutive α-helices situates R118 and R122 in positions to participate in acceptor–substrate binding of the other protomer, and produces a wide positively charged surface ( Supplementary Figs S3a and S5a ). W133 exits in dimer interface on α2 and, interestingly, W133A mutant appeared to exist as monomer in solution based on the gel filtration chromatography result ( Supplementary Fig. S4a ). Moreover, W113A mutant showed a significant decrease in sulfotransferase activity compared with the wild-type enzyme ( Fig. 2c ). These results indicate that while dimerization of TPST2 is not essential for catalysis, it does have some role in substrate binding. Comparison with other sulfotransferases and catalytic mechanism of TPST2 As with TPST2, heparan sulphate sulfotransferases, including 3- O -sulfotransferase isoform 3 (HS3OST3) [23] , are type II transmembrane Golgi-associated enzymes. Cytosolic sulfotransferases (SULTs), for example, mouse SULT1D1 (ref. 24 ), differ from their Golgi-associated counterparts in that they are soluble enzymes and recognize low-molecular-weight compounds, such as hydrophobic steroid and xenobiotics, as acceptor substrates. Structural comparisons of TPST2ΔC18 with HS3OST3 and SULT1D1 show a root mean squared deviation (r.m.s.d.) of 2.9 Å for 167 structurally equivalent Cαs and 2.8 Å for 162 structurally equivalent Cαs, respectively, but with only low sequence identities (19.1% and 14.8%, respectively). Particularly, the core elements including the 5′-PSB and 3′-PB motifs, which are involved in the binding to PAPS, are structurally conserved ( Supplementary Fig. S3a–c ). Superposition of TPST2ΔC18 with the active site of SULT1D1 complexed with PAPS and p -nitrophenol ( p NP; yellow) and that of HS3OST3 complexed with PAP and tetrasaccharide (cyan) shows that residues involved in catalytic reaction are also structurally conserved. This superposition revealed the catalytic functions of residues R78, E99, K158 and S285 of TPST2ΔC18 ( Fig. 3a , Supplementary Fig. S3a ). In the HS3OST3 structural study, E184 was proposed to serve as a catalytic base, deprotonating the 3-OH group of the glucosamine unit (GlcN) of tetrasaccharide for nucleophilic attack on the sulphonate group. A structurally equivalent E99 is present in TPST2ΔC18. The mutation of this residue resulted in a complete loss of sulfotransferase activity for mutated TPST2 ( Fig. 3b ), suggesting that E99 is indeed critical for the catalytic function of TPST2. R78 and S285 contact the bridge oxygen of the leaving phosphate group of PAP in TPST2ΔC18 structure. R78 of TPST2ΔC18 superimposes very well with K48 of SULT1D1 and K162 of HS3OST3, which were proposed to act as possible proton donors in catalysis and stabilize the transition state [25] . Interestingly, the R78A mutant displayed significantly reduced enzymatic activity ( Fig. 3b ). S285 of TPST2ΔC18 is at the equivalent position as K368 of HS3OST3. The mutation of K368 nearly abolished sulfotransferase activity for the mutated HS3OST3. The corresponding lysine residue of the N -sulfotransferase domain of N -deacetylase/ N -sulfotransferase-1 (ref. 26 ), and other heparan sulphate sulfotransferases, has been proposed to have a significant role in catalysis, but detail of its catalytic role is unknown. The S285A mutant abolishes sulfotransferase activity completely for the mutated TPST2 ( Fig. 3b ). Sasaki et al . [27] reported that H266Q mutant of mouse TPST lost catalytic activity. H267, a corresponding resiude in hTPST2, interacts with backbone carbonyl oxygen of V289 of α13. The above-mentioned S285 is present immediately before α13. Therefore, this latter interaction seems to contribute to placing S285 in its correct position for catalysis. K158 of TPST2ΔC18 superimposes with K106 of SULT1D1 and K215 of HS3OST3. The lysine residue at this position has been proposed to function in the stabilization of the transition state. Interestingly, K158A mutation significantly reduced the enzymatic activity for the mutated TPST2 ( Fig. 3b ). In addition, the positions of acceptor hydroxyl groups of all three substrates (red dashed circles in Fig. 3a ) and the 5′-phosphates of PAP/PAPS molecules are also well superimposed ( Fig. 3a ). The hydroxyl group of Y acceptor is located 2.6 Å from the sulphur atom of PAPS in SULT1D1 structure and this hydroxyl group is in a proper position for in-line nucleophilic attack as previously proposed for other sulfotransferases ( Fig. 3a ). Taken together, the transfer reaction of TPST has been proposed to proceed through an S N 2-like in-line displacement in a sequential mechanism, in which R78, E99, K158, S285 have critical roles in catalysis. R78 is a catalytic acid and E99 is a catalytic base. K158 and S285 are residues for stabilization of the transition state. Previously, a ping-pong mechanism using a His residue as a catalytic residue was proposed [28] . However, our structural and mutational studies, plus the absence of a His residue in the active site of the TPST2ΔC18 structure, strongly support a sequential mechanism. Moreover, it has been reported that Mn 2+ ion influenced the activity of TPST [16] . However, although our crystallization conditions included Mn 2+ ion, we were unable to identify its position in the structure. 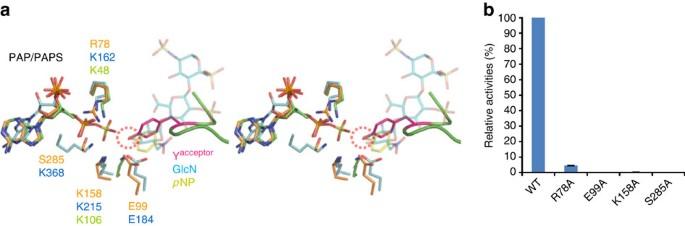Figure 3: Superposition of the catalytic sites of TPST2ΔC18, SULT1D1 and HS3OST3. (a) Stereo figure of superposition of TPST2ΔC18 with the active site of SULT1D1 complexed with PAPS andp-nitrophenol (pNP; yellow) and that of HS3OST3 complexed with PAP and tetrasaccharide (cyan). Red dashed circles indicate the positions of the three acceptor hydroxyl groups of substrates. (b) Site-directed mutagenesis experiments were performed to probe the role of specific amino-acid residues in the catalysis of TPST2. Sulfotransferase activity assay was performed using C4P5Y3 as the substrate peptide. The blue bar graph illustrates the relative activities of different mutant TPST2s, compared with that of the wild-type TPST2 as 100%.n=3, mean±s.e.m. Figure 3: Superposition of the catalytic sites of TPST2ΔC18, SULT1D1 and HS3OST3. ( a ) Stereo figure of superposition of TPST2ΔC18 with the active site of SULT1D1 complexed with PAPS and p -nitrophenol ( p NP; yellow) and that of HS3OST3 complexed with PAP and tetrasaccharide (cyan). Red dashed circles indicate the positions of the three acceptor hydroxyl groups of substrates. ( b ) Site-directed mutagenesis experiments were performed to probe the role of specific amino-acid residues in the catalysis of TPST2. Sulfotransferase activity assay was performed using C4P5Y3 as the substrate peptide. The blue bar graph illustrates the relative activities of different mutant TPST2s, compared with that of the wild-type TPST2 as 100%. n =3, mean±s.e.m. Full size image The shape of acceptor–substrate binding site and the mode of acceptor–substrate binding for these three sulfotransferases are totally different ( Supplementary Fig. S3a–c ). However, the residues involved in the acceptor–substrate binding mainly lie in the regions following 5′-PBS and 3′-PB in all three structures ( Supplementary Fig. S3a–c ). SULT1D1 takes small phenolic compounds of substrate into its hydrophobic substrate-binding site using a gate-like structure formed by two phenylalanine resides ( Supplementary Fig. S3b ). In contrast, HS3OST3 uses a widely open groove for binding to the sugar chain of substrate compounds forming many hydrogen bonds ( Supplementary Fig. S3c ). Different from these two enzymes, TPST2ΔC18 utilizes a deep narrow cleft formed by the dimer interface in substrate binding ( Supplementary Figs S3a and S5 ). The above-mentioned comparison reveals that acceptor substrates were recognized differentially by the corresponding regions around PAPS-binding motifs in three different types of sulfotransferases. Substrate peptide binding In both protomers, the bound C4P5Y3 peptide adopts an L-shaped conformation (flexed to an 86-degree angle at −1 position; Fig. 4a and Supplementary Fig. S6 ). Although each protomer binds the C4P5Y3 peptide in a slightly different manner, the interaction pattern and the structure of the E −2 -D −1 -Y acceptor -E +1 region are virtually identical between C4P5Y3 A and C4P5Y3 B . All conserved interactions with C4P5Y3 between protomer A and B are shown in Fig. 4a–c . The backbone of Y acceptor is recognized by a loop following the 3′-PB motif (backbone of Thr198-Ala200) as a short parallel β-strand (βe) ( Fig. 4a–c ). Additionally, backbone atoms at −2 to −1 position are recognized by side chains of R101 and T198. The results obtained with the T198A TPST2 mutant showing some decrease in sulfotransferase activity ( Fig. 4d ) suggested that the T198 recognizes the backbone at −1 position. Although R101A is a monomeric mutant ( Supplementary Fig. S4a ), the decrease in sulfotransferase activity of the R101A mutant was higher than that of another monomeric mutant W113A ( Fig. 2c ). These results indicate that the recognition of backbone carbonyl oxygens of E −2 and D −1 of C4P5Y3 by R101 has some role in substrate binding. The side chain of E −2 forms no interactions ( Fig. 4b ). This finding is consistent with previous studies suggesting that the residue at −2 position in substrate peptide interacts with TPST using the peptide backbone [29] , [30] . Previous studies showed, no general consensus sequence for tyrosine sulfation sites [17] , [18] . The substrate peptide backbone recognitions by TPST2 as mentioned above seem to have an important role in substrate peptide binding. 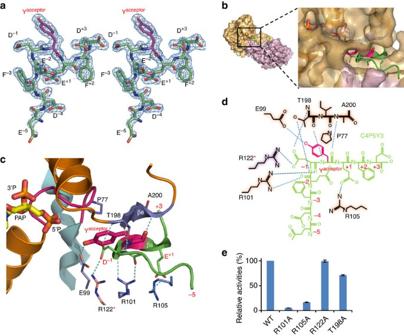Figure 4: Accepter peptide-binding site of TPST2ΔC18. (a) The electron density maps showing the stereo image of bound C4P5Y3Apeptide (simulated annealed omit Fo–Fc map contoured at 3σ). The acceptor tyrosine residue is coloured magenta. (b) Close-up views of the binding sites of C4P5Y3A(green) with surface representation. (c) Close-up views of the binding sites of C4P5Y3A(green). The interactions, in which the binding modes of TPST2ΔC18 for the peptides are identical between two active sites in the dimer, are shown. Residues of protomer A that are involved in binding to C4P5Y3Aare coloured slate blue. R122* of protomer-B, which is involved in binding to C4P5Y3A, is coloured light pink. (d) Schematic representation of conserved interaction pattern of the TPST2ΔC18 with C4P5Y3. (e) Site-directed mutagenesis experiments were performed to probe the role of specific amino-acid residues in the peptide binding of TPST2. Sulfotransferase activity assay was performed using C4P5Y3 as the substrate peptide. The blue bar graph illustrates the relative activities of different mutant TPST2s, compared with that of the wild-type TPST2 as 100%.n=3, mean±s.e.m. Figure 4: Accepter peptide-binding site of TPST2ΔC18. ( a ) The electron density maps showing the stereo image of bound C4P5Y3 A peptide (simulated annealed omit Fo–Fc map contoured at 3σ). The acceptor tyrosine residue is coloured magenta. ( b ) Close-up views of the binding sites of C4P5Y3 A (green) with surface representation. ( c ) Close-up views of the binding sites of C4P5Y3 A (green). The interactions, in which the binding modes of TPST2ΔC18 for the peptides are identical between two active sites in the dimer, are shown. Residues of protomer A that are involved in binding to C4P5Y3 A are coloured slate blue. R122* of protomer-B, which is involved in binding to C4P5Y3 A , is coloured light pink. ( d ) Schematic representation of conserved interaction pattern of the TPST2ΔC18 with C4P5Y3. ( e ) Site-directed mutagenesis experiments were performed to probe the role of specific amino-acid residues in the peptide binding of TPST2. Sulfotransferase activity assay was performed using C4P5Y3 as the substrate peptide. The blue bar graph illustrates the relative activities of different mutant TPST2s, compared with that of the wild-type TPST2 as 100%. n =3, mean±s.e.m. Full size image The phenolic hydroxyl group of the Y acceptor is hydrogen bonded to E99 and the aromatic ring forms a hydrophobic interaction with P77 of the 5′-PSB motif. A previous study indicated that the binding of TPST to a substrate peptide was enhanced in the presence of PAP [13] . This finding could be explained by the structural feature that the P77 is within the 5′-PSB motif and that βe lies in the loop following the 3′-PB motif. Therefore, it can be postulated that PAP binding not only stabilizes 5′-PSB and 3′-PB regions but also forms the peptide-binding site. Previous studies indicated that removal of the negative charge at −1 position of C4P5Y3 (cf. the D −1 -to-N mutant) led to a 20-fold increase in the K m value [19] . In the TPST2ΔC18 crystal structure, the D −1 of C4P5Y3 interacts with the side chain of R122 from the other protomer and the backbone amide nitrogen of T198 ( Fig. 4b ). The result obtained with the R122A TPST2 mutant showing little effect on the sulfotransferase activity ( Fig. 4e ) suggested that the negative charge of D −1 is specifically recognized by the backbone amide nitrogen of T198 ( Fig. 4c ). The side chain of E +1 of C4P5Y3 is hydrogen bonded to R105 of TPST2. The results obtained with the R105A mutant showed a significant decrease in the sulfotransferase activity ( Fig. 4d ). These results indicate that the interaction contributes significantly to C4P5Y3 binding. However, as the negatively charged residue at +1 position of peptide substrates is not highly conserved, this side-chain interaction is likely not common for substrate peptide binding in TPST2. The peptide-binding area is widely positively charged due to the presence of a number of arginine and lysine residues (R101, R105, K115, R118, R122, K164, K216 and R284; Supplementary Fig. S5a ) and can thus accommodate negatively charged substrates that contain tyrosine residues adjacent to several acidic residues located within −5 to +5 positions. As described above, mutational analysis showed that only two residues (R101 and R105) have some role in the recognition of C4P5Y3 ( Fig. 4d ) and all other residues are dispensable in terms of the recognition of C4P5Y3 ( Supplementary Fig. S5b ). It is possible, however, that these dispensable residues may have a role in the recognition of other protein substrates with acidic residues at the −5 to +5 position. It is to be pointed out that the original sequence of the C4P5Y3 peptide in complement C4 contains Tyr residues at the −3 and +2 positions. If Tyr residues are modelled back at these positions, the phenolic oxygen atoms in the −3 and +2 positions seem to form hydrogen bonds to R105 and R122, respectively. This latter finding indicates that Tyr residues in −5 to +5 position in the substrate sequence may contribute substrate recognition. TPSTs are enzymes responsible for the addition of a sulphonate group to tyrosine residues of target proteins during their post-translational modification. Protein tyrosine sulfation has an important role in extracellular protein–protein interactions implicated in, for example, inflammation, haemostasis and viral infection. In this study, we solved the crystal structure of TPST2ΔC18, a core domain of human TPST2, complexed with C4P5Y3, a peptide derived from complement C4, and PAP at 1.9 Å resolution. Structural analysis indicated that TPST2ΔC18 is similar in terms of the catalytic mechanism to other types of sulfotransferases, but differ substantially in the substrate recognition mode. This study demonstrated that TPST2 have four key features with regard to substrate peptide/protein recognition. First is that TPST2 can specifically recognize acceptor tyrosine on substrate proteins/peptides. This specific recognition is mediated by hydrogen bond interaction by Glu and hydrophobic interaction by Pro ( Fig. 4c ). Second is that TPST2 also recognizes backbone atoms of substrate proteins/peptides by two residues and β-sheet formation. The backbone atoms at −2 and −1 positions in the bound peptide are recognized by Arg and Thr of TPST2 and the backbone atoms of the acceptor tyrosine are recognized via a short parallel β-sheet type interaction ( Fig. 4c ). Third is that the bound substrate peptide binds in a deep cleft of TPST2ΔC18 and Y acceptor on substrate peptide is placed deep in the active site of TPST2 ( Fig. 4b ). To access the deep active site, the vicinity of the accepter Tyr residue in the substrate proteins should probably take on an intrinsically unfolded conformation. Recently, Huang et al . [31] reported that the coil structure contribute to sulfation site recognition. Thus, the majority of the sequences encompassing the accepter Tyr residue may be highly solvent-exposed and therefore are flexible and can easily adjust to the binding cleft of the TPSTs. Fourth is that TPST2 has many positively charged residues in its substrate-binding site and can recognize acidic residues within −5 to +5 position of the acceptor Tyr ( Supplementary Fig. S5a ). Taken together, an essential requirement for the substrate is that the acceptor tyrosine residue would have to be located in an intrinsically flexible region to fit into the deep cleft of hTPST2. Many electrostatic interactions are utilized in diverse substrate amino-acid sequences around tyrosine sulfation sites of proteins. 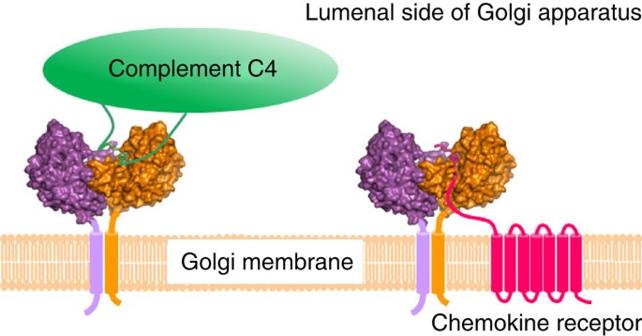Figure 5: Proposed model for the sulfation of soluble and membrane protein by TPST. The figure shows a schematic diagram illustrating the sulfation of the soluble complement C4 protein (green) and membrane-bound chemokine receptor protein (red) in the Golgi apparatus. Figure 5 shows a model for the sulfation of the soluble complement C4 protein and the membrane-bound chemokine receptor by hTPST2 in the Golgi lumen. Figure 5: Proposed model for the sulfation of soluble and membrane protein by TPST. The figure shows a schematic diagram illustrating the sulfation of the soluble complement C4 protein (green) and membrane-bound chemokine receptor protein (red) in the Golgi apparatus. Full size image To further address the substrate recognition of hTPST2, we reviewed the correlation between substrate sequences and their K m values. In a previous study, we determined kinetic constants for the TPST-mediated sulfation of various substrate peptides [16] . The tested peptide substrates can be divided into three groups based on their K m values (low, moderately high and high). The first group (including complement C4, PSGL-1 and CCR2 peptides) with low K m values contains D −1 and an acidic residue at +1 position ( Supplementary Fig. S7 ). The second group (including CCR8 and CCK) with moderately high K m values contain D −1 , but no acidic resiude at +1 position ( Supplementary Fig. S7 ). The third group (including CCR3 and CCR5) with high K m values does not contain D −1 ( Supplementary Fig. S7 ). The differences in K m values can therefore be correlated with the existence of D −1 and an acidic resiude at +1 position. As already discussed in the TPST2ΔC18 crystal structure complexed with C4P5Y3, D −1 and E +1 in C4P5Y3 are specifically recognized by the backbone amide nitrogen of T198 and side chain of R105, respectively ( Fig. 4c ). Therefore, these two interactions are main determinants for the K m values for substrate peptides. The conformations of C4P5Y3 A and C4P5Y3 B peptides are identical in the E −2 -D −1 -Y acceptor -E +1 region but divergent in the distal regions (E −5 -D −4 -F −3 and F +2 -D +3 ; Supplementary Fig. S6 ). The distal regions do not have conserved interactions between C4P5Y3 and protomer A or B ( Fig. 4c ). The side chains of E −5 , D −4 , F −2 and D +3 in the peptides are exposed to solvent, indicating residues at these positions are unconstrained. In line with this postulation, residues at these positions have been shown to be unconserved [31] . For example, CCK peptide contains a positively charged Arg at −2 position and various residues at +3 position ( Supplementary Fig. S7 ). To further elucidate the mechanism underlying substrate recognition by TPST, we will need to determine additional TPST structures complexed with other peptide substrates. In humans, there are two isoforms of TPST (TPST1 and TPST2) and these two isoforms have slightly different substrate specificities [16] . Comparison between human TPST1 and TPST2 showed that while the majority of the residues, which constitute the substrate-binding region are conserved ( Supplementary Fig. S5c ), several residues are not. These variations may therefore dictate the slight difference in substrate specificity between TPST1 and TPST2, and explain how they may accommodate a variety of substrate proteins. A surprising, yet interesting, finding is that the mode of recognition for substrate peptide observed in the TPST2ΔC18 structure seems to resemble that observed for the receptor type tyrosine kinases (IRK) [32] ( Fig. 6 ), particularly in regard to the following three points: (i) β-sheet formation (parallel or anti-parallel), (ii) hydrophobic interaction between phenol ring of target Tyr residue and Pro residue of the enzyme and (iii) hydrogen bond formation between phenolic oxygen of the target Tyr reside and acidic residue (Asp or Glu) of the enzyme. The intracellular locations of these two types of enzymes are different (Golgi lumen versus cytosol) and their substrate proteins also do not overlap. It is possible that the similarity between these two types of enzymes with regard to their peptide substrate recognition may be the result of convergent evolution, as they are both involved in the post-translational protein modification on Tyr residues. 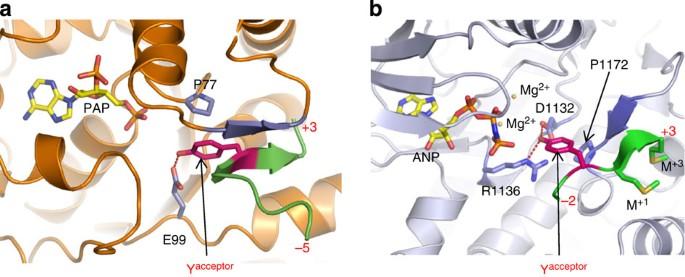Figure 6: Similarity between TPST2 and tyrosine kinase. (a) The active site of a ternary complex of TPST2ΔC18. Yacceptorresidue of the substrate peptide is coloured magenta and the rest is coloured green. The PAP is coloured yellow. Important residues for Yacceptorrecognition are coloured slate blue. (b) The active site of a ternary complex of insulin receptor tyrosine kinase (IRK, PDB id code 1IR3). Yacceptorresidue of the substrate peptide is coloured magenta and the rest is coloured green. The donor ATP analogue ANP is coloured yellow. Important residues for Yacceptorrecognition are coloured slate blue. Figure 6: Similarity between TPST2 and tyrosine kinase. ( a ) The active site of a ternary complex of TPST2ΔC18. Y acceptor residue of the substrate peptide is coloured magenta and the rest is coloured green. The PAP is coloured yellow. Important residues for Y acceptor recognition are coloured slate blue. ( b ) The active site of a ternary complex of insulin receptor tyrosine kinase (IRK, PDB id code 1IR3). Y acceptor residue of the substrate peptide is coloured magenta and the rest is coloured green. The donor ATP analogue ANP is coloured yellow. Important residues for Y acceptor recognition are coloured slate blue. Full size image To summarize, the molecular description of the TPST2ΔC18 crystal structure provides a framework for understanding the reaction mechanism of protein tyrosine sulfation, which is one of the major post-translational protein modifications. Cloning, expression and purification To circumvent potential complications associated with the crystallization of membrane proteins, we opted to express the proposed catalytic domain of TPST2 (Gly43-Ser377) that lacks the N-terminal tail, the transmembrane domain and part of the stem region. A complementary DNA (cDNA) encoding Gly43-Ser377 of TPST2 was PCR-amplified using a previously prepared pcDNA3-TPST-2 as the template [16] . The amplified cDNA was subcloned into pET15b (Novagen), which provided an N-terminal 6xHis tag and a thrombin-recognition site. The plasmid construct (designated pET15b-TPST2) thus prepared was sequenced to confirm the reading frame and fidelity of the coding region using the service of the Research Support Center, Graduate School of Medical Sciences, Kyushu University. Recombinant protein was expressed in E. coli BL21 (DE3) RIL cells (Novagen) overnight at 37 °C. The cells were collected by centrifugation, resuspended in lysis buffer (containing 50 mM Tris, pH 8.0, and 500 mM NaCl) and disrupted by sonication. The crude homogenate thus prepared was subjected to centrifugation at 12,000 g for 20 min and the pelleted fraction was resuspended in 1 M glucose solution, followed by centrifugation at 12,000 g for 20 min. The pellet was resuspended in 1% (v/v) Triton X-100 solution containing 10 mM EDTA, and centrifuged at 12,000 g for 20 min. Afterwards, TPST2 was extracted from the pellet using an extraction buffer (containing 8 M urea, 50 mM Tris-HCl, pH 8.0, and 500 mM NaCl) at 10 °C for 1 h. The extracted fraction was centrifuged at 12,000 g for 30 min. The supernatant collected was applied to a Ni-NTA agarose gel (Qiagen) column, and the bound TPST2 was eluted from the column using the above-mentioned extraction buffer supplemented with 200 mM imidazole. Refolding of the TPST2, thus purified, was performed based on a method modified from a previously reported slow dialysis protocol [33] . Afterwards, the buffer was exchanged with a binding buffer (containing 50 mM Tris-HCl, pH 7.0, and 100 mM NaCl) using a Sephadex G-25 (GE Healthcare) buffer-exchange column. TPST2 thus prepared was further purified using a Resource S (GE Healthcare) cation-exchange column. Bound proteins were eluted using a linear gradient (from 0.1 to 1 M) of NaCl, and the eluent was monitored by A280 nm. The purified soluble form of TPST2 was incubated with trypsin (Sigma) overnight at 10 °C, and the resulting proteolytically defined TPST2, a 38-kDa core domain of TPST2 (TPST2Δ18), was sequenced to show that it corresponds to the Gly43-Leu359 region of TPST-2. A cDNA encoding Gly43-Leu359 (TPST2ΔC18) was subcloned into pET15b (Novagen). The plasmid construct (designated pET15b-TPST2ΔC18) was sequenced to confirm the reading frame and fidelity of the coding region. Bacterial expression and purification of the recombinant TPST2ΔC18 was performed using the same protocol for the recombinant TPST2 as described above. Purified TPST2ΔC18 was concentrated by ultrafiltration to a concentration of 2 mg ml −1 . To the concentrated TPST2ΔC18 solution, PAP, MnCl 2 and the C4P5Y3 peptide were added to final concentrations of 5, 1 and 1 mM, respectively. Crystallization and data collection Crystals of TPST2ΔC18 were prepared by using the sitting-drop vapour-diffusion method at 20 °C. The sitting drop contained 100 nl of the above-mentioned TPST2ΔC18 preparation mixed with 100 nl of a reservoir solution consisting of 0.1 M sodium malonate (pH 5.0), and 10–12% polyethylene glycol 3350. For data collection, crystals were transferred to a cryo buffer (0.1 M sodium malonate, pH 5.0, 10–12% polyethylene glycol 3350, 50 mM Tris-HCl, pH 7.0, 200 mM NaCl, 5 mM PAP, 1 mM MnCl 2 , 5 mM C4P5Y3 peptide and 10% glycerol). Thereafter, the preparation was flash frozen using a cryo system (Rigaku). A 1.9-Å resolution data set was collected at beamline BL5A, Photon Factory, Tsukuba, JAPAN. The structure of TPST2ΔC18-PAP-C4P5Y3 complex was solved by single isomorphous replacement and anomalous scattering using an iodide derivative. TPST2ΔC18-PAP-C4P5Y3 crystals were soaked for 30 s in a cryo buffer containing 1 M potassium iodide and thereafter the preparation was flash frozen using a cryo system (Rigaku). A 22.1-fold redundant 2.0-Å data set was collected at beamline BL38B1, SPring-8, Hyogo, Japan. For TPST2-PAP binary complex, PAP and MnCl 2 were added to final concentrations of 5 mM and 1 mM, respectively. Crystals of TPST2 were grown by using the sitting-drop vapour-diffusion method at 20 °C. The sitting drop contained 100 nl of purified TPST2 solution mixed with 100 nl of a reservoir solution consisting of 0.1 M Tris-HCl, pH 7.0, 0.1 M calcium acetate and 20% polyethylene glycol 3000. For data collection, crystals were transferred to a solution containing 0.1 M Tris-HCl, pH 7.0, 0.1 M calcium acetate, 20% polyethylene glycol 3000, 50 mM Tris-HCl, pH 7.0, 200 mM NaCl, 5 mM PAP, 1 mM MnCl 2 and 10% glycerol. Thereafter, the preparation was flash frozen in liquid nitrogen. A 3.5-Å resolution data set was collected at beamline BL17A, Photon Factory, Tsukuba, Japan. Structure solution and refinement The initial phase of the structure determination of the TPST2ΔC18-PAP-C4P5Y3 complex was performed using the native and iodide derivative data with the program package HKL2MAP [34] . The density modification was applied to the initial phase using RESOLVE [35] . The partial model was built automatically using RESOLVE and ARP/wARP [36] , and modified manually using COOT [37] . The structure was revised several times by alternately adjusting the model and refinements using Refmac [38] . Refinement statistics are summarized in Table 1 . Structure quality was assessed using PROCHECK [39] . Table 1 Data collection, phasing and refinement statistics. Full size table The structure of PAP-bound form of TPST2 was solved by molecular replacement using the coordinates of TPST2ΔC18-PAP-C4P5Y3 dimer as a search model and the program Phaser [40] as a tool. The structures were revised several times by alternately adjusting the model and refinements using COOT and Refmac. Refinement statistics are summarized in Table 1 . Structure quality was assessed using PROCHECK. Mutational analysis pET15b harbouring cDNAs encoding TPST2 mutants were prepared using the PCR-based Takara PrimeSTAR mutagenesis basal kit, with pET15b-TPST2 as the template, based on the protocol recommended by the manufacturer. The primers used for the PCR amplification of the mutants were synthesized by Sigma-Genosys. The PCR-amplified pET15b-TPST2 mutant constructs were sequenced to confirm the anticipated mutations using the service of the Research Support Cenetr, Graduate School of Medical Sciences, Kyushu University. TPST2 wild type and mutants for mutational analysis were expressed in Origami (DE3) cells (Novagen) carrying pGro7 (Takara, Japan) plasmids encoding chaperonin proteins GroEL and GroES. Upon an overnight induction at 30 °C, the cells were collected by centrifugation at 5,000 g for 20 min, resuspended in lysis buffer and disrupted by sonication. The crude homogenate thus prepared was subjected to centrifugation at 12,000 g for 20 min, and the supernatant was applied to a Ni-NTA agarose column. The bound proteins were eluted from the column using the lysis buffer containing 200 mM imidazole. DTT (at the final concentration of 1 mM) was added to the eluted fraction, and the TPST2 therein was concentrated by centrifugal filters (Amicon Ultra 3K, Millipore), and further purified using a Superdex 200 16/60 (GE Healthcare) column. The eluted fractions containing TPST2 mutant protein were pooled. The buffer was exchanged with a new buffer (containing 50 mM Tris-HCl, pH 7.0, and 150 mM NaCl) using a Sephadex G-25 buffer-exchange column. The purity of the TPST2 mutant protein thus prepared was confirmed by 12.5% SDS–PAGE. The sulfotransferse activity assays of wild-type and mutant TPST2s were performed as described previously [16] . Accession codes: Structure factors TPST2ΔC18-PAP-C4P5Y3 and TPST2-PAP have been deposited in the Protein Data Bank under accession numbers 3AP1 and 3AP3 , respectively. How to cite this article: Teramoto, T. et al . Crystal structure of human tyrosylprotein sulfotransferase-2 reveals the mechanism of protein tyrosine sulfation reaction. Nat. Commun. 4:1572 doi: 10.1038/ncomms2593 (2013).